Actin-based confinement of calcium responses duringShigellainvasion Shigella , the agent of bacillary dysentery, invades epithelial cells by locally inducing actin reorganization. Upon cell invasion, Shigella induces calcium (Ca 2+ ) signalling, but its role in invasion has remained unclear. Here we show that components involved in inositol 1, 4, 5- trisphosphate (InsP 3 ) signalling are implicated in Shigella invasion. Although global Ca 2+ responses are dispensable for bacterial invasion, local Ca 2+ responses of unprecedented long duration are associated with invasion sites. Fluorescence recovery after photo-bleaching experiments indicate that diffusion of small solutes is hindered at Shigella -invasion sites and that diffusion hindrance is dependent on bacterially induced actin reorganization. Computational simulations and experimental challenge of the model support the notion that local accumulation of InsP 3 permitted by restricted diffusion and enrichment of InsP 3 receptors account for sustained local Ca 2+ increases at entry sites. Thus, cytoskeletal reorganization through diffusion hindrance shapes the duration of local Ca 2+ signals. Upon ingestion, Shigella invades the colonic mucosa where it elicits an intense inflammatory reaction leading to tissue destruction [1] , [2] , [3] . The virulence of Shigella depends on a type III secretion system (T3SS), which injects bacterial effectors into target cells [4] . The T3SS is inactive under basal conditions, but upon cell contact, secretes two hydrophobic substrates, IpaB and IpaC, which insert into host cell membranes, forming a ‘tranlocator’ required for the injection of T3SS effectors. Cytoskeletal reorganization by these effectors lead to bacterial invasion, a process that implicates a coordination of RhoGTPases and tyrosine kinase signalling at the membrane [3] , [5] . In addition to its role in T3SS effector translocation, IpaC also induces actin polymerization responsible for the formation of cell extensions that surround the bacterium [6] . Actin polymerization at entry sites is favoured by IpgB1, a Shigella T3S-injected effector, that recruits ELMO/Dock180 and amplifies membrane rufflings at bacterial entry sites [7] . IpaA binds to the focal adhesion protein vinculin and triggers bacterial anchorage in bacterially induced actin foci, as well as the depolymerization of actin required for efficient invasion [3] , [8] , [9] . Shigella invasion also triggers global Ca 2+ responses implicated in the opening of connexin hemichannels and cell–cell signalling dependent on ATP release [10] . Hemichannel-mediated signalling favours bacterial invasion and dissemination across the epithelial layer, and participate in the induction of water release by colonocytes during in vivo infection of mice with Citrobacter rodentium [10] , [11] . Many bacterial pathogens perturb global cell Ca 2+ homoeostasis, either through secreted bacterial toxins or during direct interactions with host cells [12] , [13] , [14] , [15] . Insertion of the T3SS translocator into host cell membranes may trigger intracellular Ca 2+ increases linked to its pore-forming activity and Ca 2+ influx, or by inducing alterations of the host plasma membranes leading to InsP 3 -dependent signalling, resulting from the mobilization of Ca 2+ from intracellular stores [16] , [17] . InsP 3 may in turn induce oscillatory patterns of global intracellular Ca 2+ in individual cells [10] , [18] , [19] . Although global Ca 2+ responses may have long-term consequences by activating gene transcription, local Ca 2+ signals, evoked by weak InsP 3 stimuli, can occur independently of global Ca 2+ increases. These Ca 2+ signals, confined in a small cytoplasmic region around the Ca 2+ -releasing sites [20] , correspond to elementary events of Ca 2+ release from discrete clusters of channels from intracellular pools [21] . Local Ca 2+ signals occuring within the vicinity of the plasma membrane could directly regulate Ca 2+ -dependent processes, including processes involving cortical actin reorganization. [22] , [23] , [24] . Here we show that InsP 3 -mediated signalling is required for Shigella invasion of epithelial cells. Shigella triggers the recruitment of InsP 3 receptors, PLC-β1 and PLC-δ1 at entry sites, shown to participate in the invasion process. Unusually long-lasting local Ca 2+ responses are correlated with restriction of diffusion linked to actin polymerization at bacterial invasion sites and the local activation of mitochondria at entry sites. Role of InsP 3 -mediated signalling during Shigella invasion We used an InsP 3 -5 phosphatase (InsP 3 -5P) expressed from a green fluorescent protein (GFP) polycistronic construct to investigate the implication of InsP 3 -mediated Ca 2+ signalling in Shigella invasion [25] . As expected, InsP 3 -5P-transfected cells did not elicit whole-cell Ca 2+ responses in response to relevant agonists or to Shigella challenge, indicating efficient inhibition of InsP 3 -mediated signalling ( Fig. 1a and Supplementary Fig. S1 ). For the pIRES-5P-GFP transfection, bacterially induced actin foci were scored in transfected cells identified using GFP fluorescence. InsP 3 -5P transfection, strikingly, led to inhibition of bacterially induced actin foci, with only 20% of foci forming per cell compared with GFP-transfected cells ( Fig. 1b and Supplementary Fig. S2 ). Consistent with the implication of InsP 3 -mediated signalling in Shigella invasion, immunofluorescence labelling indicated that InsP 3 -R type 1 (InsP 3 R1) and type 3 (InsP 3 R3), the main InsP 3 Rs expressed in HeLa cells [26] , were recruited at bacterially induced actin foci, although recruitment appeared less consistent for InsP 3 R3 ( Supplementary Fig. S3 ). In contrast, an ER-YFP probe and anti-calnexin staining did not show particular enrichment at Shigella -invasion sites ( Supplementary Fig. S3 ). To confirm the implication of InsP 3 -mediated signalling in Shigella invasion, we used siRNAs directed against InsP 3 Rs. As previously described, inhibition of InsP 3 Rs expression impaired Ca 2+ responses upon agonist stimulation [26] ( Supplementary Fig. S4 ). Consistent with results obtained with the InsP 3 -5P, bacterially induced actin foci formation was depressed in cells treated with anti-InsP 3 Rs siRNAs, with a 68% inhibition compared with control cells ( Fig. 1c ). 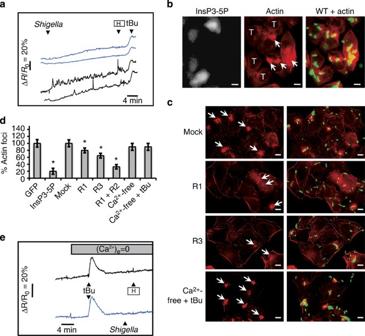Figure 1: InsP3-mediated signalling is required forShigella-induced actin foci formation. Variations of global intracellular Ca2+in HeLa cells transfected with the InsP3-5P (blue), or GFP (black), challenged with wild-type (WT)Shigellain EM buffer (a), or in Ca2+-free medium (e). H, addition of histamine at a 30 μM final concentration. Cells tested did not show any Ca2+response when stimulated with histamine 100 μM final concentration or followingShigellainfection. (b,c) Cells challenged with invasiveShigellalabelled by anti-lipopolysaccharide staining (green) and F-actin (red). Arrows: actin foci. (b) T, cells transfected with InsP3-5P. (c) Cells mock-transfected, transfected with siRNAs against InsP3R1 (R1) or InsP3R3 (R3), or incubated in Ca2+-free buffer and stimulated with tBuBHQ (Ca2+-free+tBu). Scale bar, 5 μm. (d) Actin foci were scored in cells labelled as inb,c, and average values±s.e.m. were expressed as a percentage of the values obtained for: GFP (129 cells,N=3) for InsP3-5P-transfected cells (129 cells,N=3); Mock-transfected cells (1,270 foci, 2,558 cells,N=4) for cells transfected with siRNAs against InsP3R1 (787 foci, 1,966 cells,N=4), InsP3R3 (730 foci, 2,298 cells,N=4), or InsP3R1 and InsP3R3 (269 foci, 1,623 cells,N=4); cells challenged in EM buffer for cells in Ca2+-free buffer or subjected to Ca2+-depletion treatment (>200 cells,N=3). *, statistical significance relative to control was tested using an unpaired Student’st-test with unequal variance.P=10−7(InsP3-5P);P=0.0142 (R1);P=0.001 (R3);P=2 × 10−5(R1+R3). Figure 1: InsP 3 -mediated signalling is required for Shigella -induced actin foci formation. Variations of global intracellular Ca 2+ in HeLa cells transfected with the InsP 3 -5P (blue), or GFP (black), challenged with wild-type (WT) Shigella in EM buffer ( a ), or in Ca 2+ -free medium ( e ). H, addition of histamine at a 30 μM final concentration. Cells tested did not show any Ca 2+ response when stimulated with histamine 100 μM final concentration or following Shigella infection. ( b , c ) Cells challenged with invasive Shigella labelled by anti-lipopolysaccharide staining (green) and F-actin (red). Arrows: actin foci. ( b ) T, cells transfected with InsP 3 -5P. ( c ) Cells mock-transfected, transfected with siRNAs against InsP 3 R1 (R1) or InsP 3 R3 (R3), or incubated in Ca 2+ -free buffer and stimulated with tBuBHQ (Ca 2+ -free+tBu). Scale bar, 5 μm. ( d ) Actin foci were scored in cells labelled as in b , c , and average values±s.e.m. were expressed as a percentage of the values obtained for: GFP (129 cells, N =3) for InsP 3 -5P-transfected cells (129 cells, N =3); Mock-transfected cells (1,270 foci, 2,558 cells, N =4) for cells transfected with siRNAs against InsP 3 R1 (787 foci, 1,966 cells, N =4), InsP 3 R3 (730 foci, 2,298 cells, N =4), or InsP 3 R1 and InsP 3 R3 (269 foci, 1,623 cells, N =4); cells challenged in EM buffer for cells in Ca 2+ -free buffer or subjected to Ca 2+ -depletion treatment (>200 cells, N =3). *, statistical significance relative to control was tested using an unpaired Student’s t -test with unequal variance. P =10 −7 (InsP3-5P); P =0.0142 (R1); P =0.001 (R3); P =2 × 10 −5 (R1+R3). Full size image Shigella invasion does not require global Ca 2+ responses To deplete cells from Ca 2+ , while limiting cytotoxic effects associated with the use of Ca 2+ chelators over the length of the expriments, cells were incubated in Ca 2+ -free medium and treated with 2, 5-di (tert-butyl)-1, 4-benzohydroquinone (tBuBHQ), an inhibitor of the sarco-endoplasmic Ca 2+ ATPase involved in the replenishing of intracellular pools, at a final concentration of 25 μM at 37 °C for 10 min ( Fig. 1e ). Under such treatment, cells did not show significant alterations of their morphology but failed to show global Ca 2+ responses when stimulated with 30 μM histamine or when challenged with Shigella ( Fig. 1e ). In contrast, following Ca 2+ depletion and tBuBHQ treatment, long-lasting local Ca 2+ responses could still be observed upon Shigella infection ( Supplementary Fig. S5 ). Although tBuBHQ treatment in Ca 2+ -free medium inhibited global Ca 2+ responses induced by Shigella , bacterially induced actin foci occurred at levels indistinguishable from untreated controls ( Fig. 1c–e ). Remarkably, when cells were treated with the Ca 2+ chelator BAPTA-AM, known to inhibit global as well as local Ca 2+ responses [20] , [21] , the average frequency of actin foci per cell decreased significantly, with only 3±1.6% observed when compared with control untreated cells ( Supplementary Fig. S6 ). Together, these results implicate InsP 3 -mediated signalling, but not global Ca 2+ responses, in Shigella -induced cytoskeletal reorganization and bacterial invasion, suggesting that local Ca 2+ signals that depend on InsP 3 synthesis participate in Shigella invasion. Local Ca 2+ responses associated with Shigella actin foci Transient and local Ca 2+ signals, remaining confined to a small cytoplasmic region at Ca 2+ -releasing sites, have been described to occur independently of global Ca 2+ responses, in association with cytoskeletal reorganization [23] , [24] . The implication of InsP 3 signalling in Shigella invasion prompted us to study local Ca 2+ responses during bacterial entry.To study local Ca 2+ responses during bacterial entry, Fluo-4-loaded cells were challenged with Shigella and subjected to high-speed fluorescence microscopy (HSFM). A major difficulty in these experiments is that, as opposed to Ca 2+ agonists, bacterial invasion does not occur in a fully synchronized manner and need to be analysed over several minutes. Because in our conditions, HSFM over prolonged acquisition was not compatible with bacterial invasion, we performed series of ‘snap-shot’ HFSM analysis at various time points following bacterial challenge. As shown in Fig. 2 , local Ca 2+ responses induced by bacterial challenge could be detected as early as 5 min following bacterial challenge, with an average duration of 100–400 ms with an increase in Ca 2+ concentration corresponding on average to 6.9% of the maximal cytosolic concentration achieved during global responses, similar to the previously described ‘puffs’ [21] , [24] ( Fig. 2a ). These ‘puff-like’ responses were induced in 30–50% of the cells challenged and observed with wild type as well as the T3SS-deficient mxiD strains, indicating that these occurred independent of invasion and were likely to be induced by bacterial adhesion onto the cell surface ( Fig. 2a ). Strikingly, however, atypical sustained local responses associated with an area larger than 10 μm 2 were specifically observed for cells challenged with invasive Shigella , but never with the non-invasive mxiD mutant strain. For the analysis, these sustained local Ca 2+ responses were arbitrarily categorized into responses lasting from 0.4 to 5 s, with increases in Ca 2+ concentration ranging from 11 to 47% of the maximal response, referred to as ‘INTs’ for ‘responses of intermediate duration’ ( Fig. 2c ), or Ca 2+ responses lasting between 5 and 20 s, called ‘RATPs’ for ‘Responses Associated with Trespassing Pathogens’, which on average corresponded to 55% of the maximal response ( Fig. 2e ). INTs and RATPs were seldom detected at 5 min following cell challenge by wild-type Shigella , but occurred with an increased frequency upon further incubation to reach 40% of cells after 15 min ( Fig. 2c ). Ratiometric measurements performed in cells loaded with a combination of Fluo-4 and Fura-red ruled out the possibility of a bias linked to accumulation of the probe in RATPs ( Supplementary Fig. S7 ). Because of their size and timing of occurence, we suspected that INTs and RATPs were associated with bacterial invasion sites. To test this, samples were visualized by phase contrast microscopy following HSFM. In all samples analysed, INTs and RATPs were always associated with bacterially induced membrane ruffles corresponding to invasion sites ( Fig. 2g and Supplementary Fig. S8 ; 363 cells, N =20). Consistently, RATPs were associated with actin-rich membrane ruffles ( Fig. 2g ). 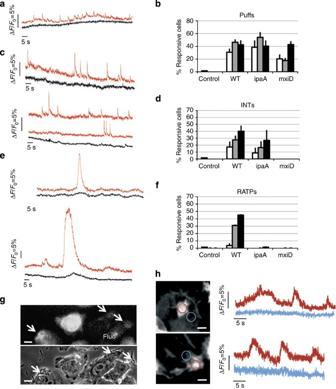Figure 2:Shigellainduces long-lasting local Ca2+responses associated with invasion sites. HeLa cells challenged withShigellastrains and analysed by HSFM. (a,c,e) Each set of traces correspond to local variations of intracellular Ca2+in the same cell. ‘Puff-like’ (a) or INT responses (c) induced byipaAmutant; (e) RATP responses induced by wild-type (WT)Shigella. (b,d,f) Percentage of cells±s.e.m showing puff (b), INT (d) or RATP (f) responses at 5 (empty bars), 10 (grey bars) and 15 min (solid bars) following bacterial challenge. Unstimulated cells (control, 37 cells,N=4), or cells challenged for 5, 10 or 15 min with WT (52, 58 and 40 cells, respectively,N=4),ipaAmutant (57, 61 and 67 cells, respectively,N=5) ormxiDmutant (44, 51 and 43 cells, respectively,N=3). (g,h) Cells challenged with WTShigella. Arrows, RATPs; (G, bottom), phase contrast; Fluo, Fluo-4 fluorescence. (h) F-actin staining (left panels) and local Ca2+responses associated with bacterially induced foci (red traces) or control area (blue traces). Scale bar, 5 μm. Figure 2: Shigella induces long-lasting local Ca 2+ responses associated with invasion sites. HeLa cells challenged with Shigella strains and analysed by HSFM. ( a , c , e ) Each set of traces correspond to local variations of intracellular Ca 2+ in the same cell. ‘Puff-like’ ( a ) or INT responses ( c ) induced by ipaA mutant; ( e ) RATP responses induced by wild-type (WT) Shigella . ( b , d , f ) Percentage of cells±s.e.m showing puff ( b ), INT ( d ) or RATP ( f ) responses at 5 (empty bars), 10 (grey bars) and 15 min (solid bars) following bacterial challenge. Unstimulated cells (control, 37 cells, N =4), or cells challenged for 5, 10 or 15 min with WT (52, 58 and 40 cells, respectively, N =4), ipaA mutant (57, 61 and 67 cells, respectively, N =5) or mxiD mutant (44, 51 and 43 cells, respectively, N =3). ( g , h ) Cells challenged with WT Shigella . Arrows, RATPs; (G, bottom), phase contrast; Fluo, Fluo-4 fluorescence. ( h ) F-actin staining (left panels) and local Ca 2+ responses associated with bacterially induced foci (red traces) or control area (blue traces). Scale bar, 5 μm. Full size image Restricted diffusion of small solutes at Shigella actin foci In other systems, the extent of diffusibility of integral membrane proteins was shown to regulate Ca 2+ signalling and phagocytic processes [27] , [28] . During Shigella invasion, the unusually long duration of RATPs suggested that diffusion of signals was restricted in the cytosolic locale corresponding to bacterial entry sites. To test this, cells were loaded with the freely diffusible dye calcein and challenged with Shigella . Bacterially induced actin foci, readily observed in calcein-loaded cells, were subjected to fluorescence recovery after photo-bleaching (FRAP) analysis and HSFM [29] ( Fig. 3a ). The diffusion rate in Shigella foci was remarkably conserved in the various determinations, with a half-maximal recovery rate t 1/2 =302±14 ms ( Table 1 and Fig. 3d ). This value was significantly higher than the t 1/2 =187±9 ms determined in control area corresponding to the free diffusion of calcein in the cell cytosol ( Table 1 ). Addition of 0.5 μM cytochalasin D or 2 μM latrunculin B, which block actin polymerization, led to the rapid disorganization of bacterially induced actin foci, with the disappearance of large actin-rich ruffles and the dense actin meshwork contacting bacteria ( Fig. 3e ). Consistent with actin filaments restricting diffusion at Shigella -invasion sites, FRAP analysis of cytochalasin D- or latrunculin B-treated foci indicated t 1/2 of 246±14 ms ( Table 1 ) and 202±10 ms (25 foci, N =3), respectively. These values were significantly lower than those obtained for foci induced by wild-type Shigella in untreated samples with P =0.0117 for cytochalasin- and P =0.0126 for latrunculin-treated cells when tested with an unpaired Student’s t -test with unequal variance. 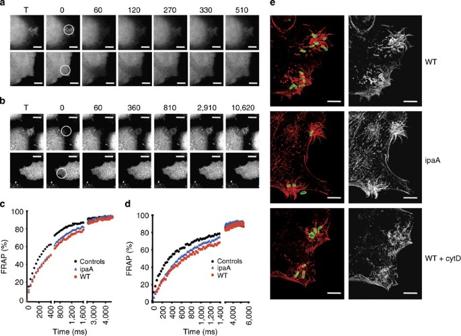Figure 3: Restriction of diffusion inShigella-invasion foci. (a–d,f) FRAP analysis ofShigella-invasion foci. (a,b) Representative time-lapse images of invasion foci (top panels) or control (bottom panels). Empty circle, bleached area. The time after bleach is indicated in ms for cells loaded with calcein (a,c) or fATP (b,d). (c,d) Fluorescence recovery kinetics in %; black, control area; foci induced by wild-type (WT)Shigella(red) oripaAmutant (blue). Broken time scales are depicted to better show differences between kinetics. (e) Staining of F-actin (red and grey levels) and bacterial lipopolysaccharide (green) of foci induced by: +CytD, with cytochalasin D; ipaA:ipaAmutant. Scale bar, 5 μm. Figure 3: Restriction of diffusion in Shigella -invasion foci. ( a – d , f ) FRAP analysis of Shigella -invasion foci. ( a , b ) Representative time-lapse images of invasion foci (top panels) or control (bottom panels). Empty circle, bleached area. The time after bleach is indicated in ms for cells loaded with calcein ( a , c ) or fATP ( b , d ). ( c , d ) Fluorescence recovery kinetics in %; black, control area; foci induced by wild-type (WT) Shigella (red) or ipaA mutant (blue). Broken time scales are depicted to better show differences between kinetics. ( e ) Staining of F-actin (red and grey levels) and bacterial lipopolysaccharide (green) of foci induced by: +CytD, with cytochalasin D; ipaA: ipaA mutant. Scale bar, 5 μm. Full size image Table 1 Half-maximal recovery values from FRAP experiments indicate restricted diffusion in Shigella -induced foci Full size table Because of the small size of the calcein tracer, its restriction of diffusion is unlikely due to a ‘sizing’ effect, but rather to a ‘crowding’ effect of the actin meshwork described elsewhere for the diffusibility of cytosolic proteins [29] , [30] , which could be viewed as a lengthening of the trajectories that have to be covered by the particles through the meshwork. Because our findings suggested that such a ‘crowding’ effect also applied to small molecules, we extended these FRAP experiments to different size fluorescent tracers. Cells were microelectroporated with fluorescent ATP (fATP), 3 or 10 kDa dextrans in cells before infection and FRAP analysis (Methods). This analysis confirmed restriction of diffusion in invasion foci, which was more pronounced with higher molecular weight tracers, with up to a 2.5-fold difference in the t 1/2 for the 10 kDa fluorescein isothiocyanate (FITC)-conjugated dextran (FITC-dextran) between entry foci compared with the cytosol control ( Table 1 , Fig. 3d and Supplementary Fig. S9 ). Shigella actin foci as local source of InsP 3 production We then investigated how actin-based diffusion hindrance could shape InsP 3 -dependent signalling and create RATPs at Shigella -invasion sites. We first wanted to determine whether Shigella -induced foci corresponded to local sources of InsP 3 production, based on the recruitment of InsP 3 -signalling component. Among the phospholipase Cs (PLCs) expressed in HeLa cells, PLC-β1 and PLC-δ1 were found to be recruited at Shigella -induced foci ( Fig. 4c , Supplementary Fig. S10 and S11 ). Cell treatment with shRNAs against PLC-β1 and PLC-δ1 resulted in a 38% decrease in foci formation, indicating their implication in Shigella -induced cytoskeletal reorganization ( Supplementary Fig. S9 ). Consistent with PLC activation and local InsP 3 production, Shigella -induced foci were strongly labelled with a GFP-PH PLC-δ1 probe for InsP 3 (ref. 31 ) ( Fig. 4b ). When quantified, the enrichment of these InsP 3 -signalling components ranged between 1.7 and 2.5 fold the average levels observed in the cell (>50 foci, N =3; Methods; Fig. 4 and Supplementary Fig. S11 ). No significant difference could be detected between enrichment observed in foci induced by wild-type Shigella and the ipaA mutant, indicating the bacterially induced InsP 3 signalling occured independent of this T3SS-injected effector ( Fig. 4a and Supplementary Fig. S11C ). Similarly, actin foci induced by other Shigella mutants deficient for the T3SS-injected invasion effectors IpaA, IpgB1 and IpgD still showed enrichment of InsP 3 R1 ( Fig. 4 and Supplementary Fig. S12 ). In contrast, such InsP 3 R1 enrichment was not observed for T3SS-deficient mxiD mutant, or translocator component-deficient ipaB or ipaC mutants ( Supplementary Fig. S12 ). These results suggested that InsP 3 Rs enrichment at bacterial invasion sites were induced by the T3SS translocator components at the plasma membrane, presumably following local activation of a PLC and InsP 3 production. Together, these data support the notion that Shigella -invasion sites correspond to local sources of InsP 3 production, enriched in InsP 3 -signalling components. 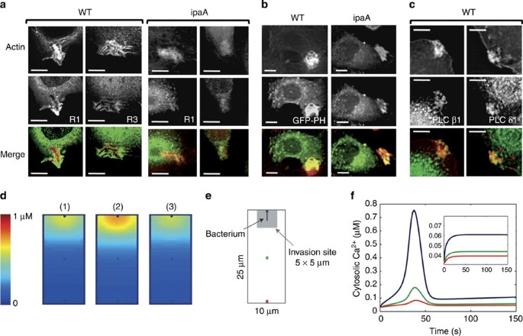Figure 4: Enrichment of InsP3-signalling components and simulations of local Ca2+increases atShigella-invasion sites. (a–c) Fluorescence micrographs of invasion foci induced by wild-type (WT)ShigellaoripaAmutant as indicated. Top panels: F-actin; middle panels: InsP3R1 (a, R1) or InsP3R3 (a, R3), GFP-PHPLC-δ1(b), or PLC-β1 (c, left), PLC-δ1’ (c, right). (d) Simulated levels of cytosolic Ca2+at 35 (1), 40 (2) and 45 s (3) after the onset of bacterial invasion depicted in colour scale with dark blue and red corresponding to 0 and 1 μM, respectively. (e) Schematic representation of the system simulated ind. For integration, the system is divided in 60 × 24 mesh points, indexed by i and j, respectively. In the region i=1–12 and j=6–19,DCandDIare divided by 1.6 andk1is multiplied by 3.JIPis equal to 15 μMs−1for i=1–7 and j=11–13, and 0 everywhere else. (f). Evolution of Ca2+concentrations at the upper (invasion site) (blue), medium (green) and lower (red) point in (1)–(3). Inset: simulations performed without restricted diffusion (see Methods). Figure 4: Enrichment of InsP3-signalling components and simulations of local Ca 2+ increases at Shigella -invasion sites. ( a – c ) Fluorescence micrographs of invasion foci induced by wild-type (WT) Shigella or ipaA mutant as indicated. Top panels: F-actin; middle panels: InsP 3 R1 ( a , R1) or InsP 3 R3 ( a , R3), GFP-PH PLC-δ1 ( b ), or PLC-β1 ( c , left), PLC-δ1’ ( c , right). ( d ) Simulated levels of cytosolic Ca 2+ at 35 (1), 40 (2) and 45 s (3) after the onset of bacterial invasion depicted in colour scale with dark blue and red corresponding to 0 and 1 μM, respectively. ( e ) Schematic representation of the system simulated in d . For integration, the system is divided in 60 × 24 mesh points, indexed by i and j, respectively. In the region i=1–12 and j=6–19, D C and D I are divided by 1.6 and k 1 is multiplied by 3. J IP is equal to 15 μMs −1 for i=1–7 and j=11–13, and 0 everywhere else. ( f ). Evolution of Ca 2+ concentrations at the upper (invasion site) (blue), medium (green) and lower (red) point in (1)–(3). Inset: simulations performed without restricted diffusion (see Methods). Full size image Modelling Shigella -induced long-lasting local Ca 2+ responses We then resorted to theoretical modelling to apprehend how, from the bacterial point source of InsP 3 synthesis, the restricted diffusion could shape localized Ca 2+ responses with long duration, such as RATPs, despite the high diffusivity of Ca 2+ and InsP 3 . We first analysed spatial inhomogeneities in InsP 3 signalling. Based on our results, we postulated that PLC activation at the site of contact between the bacterium and the cell plasma membrane stimulated localized InsP 3 synthesis in a 2.5 × 1.2 μm 2 region inside the actin focus, represented as a 5 × 5 μm 2 region in the simulated 25 × 10 μm 2 cell ( Supplementary Fig. S13A ). We assigned a value for the InsP 3 diffusion coefficient 1.6 times lower in the actin focus than in the remaining cytoplasm. This 1.6 times decrease in the diffusion coefficient at bacterial invasion sites was based on the value that we determined for the freely diffusible dye calcein, and may correspond to an underestimation of the decreased diffusibility of InsP 3 , likely to be further restricted by interactions with InsP 3 -signalling components observed in Fig. 4a–c . Indeed, fATP, which may present diffusion characteristics closer to those of InsP 3 , showed a 1.8 decrease in diffusion in Shigella -invasion sites compared with the control cell area. Our simulations, taking into account a stimulated rate of InsP 3 synthesis of 15 μMs −1 and the 1.6-fold restriction of diffusion observed at Shigella -invasion sites, indicated the presence of a gradient of InsP 3 from the source of PLC-activation site corresponding to the bacterial site of contact with the cell membrane. This gradient was maintained throughout the duration of InsP 3 synthesis ( Supplementary Fig. S13B ). According to the model, a modest gradient in InsP 3 concentration resulted in a pronounced gradient in Ca 2+ release when combined to the observed accumulation of InsP 3 receptors at the invasion site ( Supplementary Fig. S13C ). This enhanced Ca 2+ release could in turn be responsible for RATPs. We thus modelled the spatio-temporal evolution of Ca 2+ concentration by simulating the activity of InsP 3 receptors and concentrations of Ca 2+ and InsP 3 [32] (Methods). Besides a classical description of InsP 3 -mediated Ca 2+ exchanges between the cytoplasm and the intracellular pools, the model took into account-specific features related to Shigella invasion: the reduced diffusivity, the higher density of InsP 3 receptors in actin foci and the stimulation of PLC activity at the invasion site. As shown in Fig. 4d–f , confined RATP-like responses lasting for up to 20 s were simulated under these conditions. The synergistic effect of reduced diffusion and receptor enrichment relied on the highly non-linear nature of InsP 3 -induced Ca 2+ release, due to its self-amplification through Ca 2+ -induced Ca 2+ release [33] . As schematized in Supplementary Fig. S13B, S13C , slight variations of InsP 3 levels were further amplified at the levels of Ca 2+ concentrations, through the inhomogeneous density of InsP 3 Rs and the intrinsic steep dependence of the activity of this channel on InsP 3 concentration ( Supplementary Fig. S13C ). This mechanism for RATPs occurrence predicted by our phenomenological model was robust with respect to changes in parameter values and in agreement with the observed absence of Ca 2+ responses in cells overexpressing InsP 3 -5 phophatase or incubated in a Ca 2+ -free medium. Simulations performed with a 1.8 instead of a 1.6 decrease in the diffusion coefficient of InsP 3 parameter led to RATPs with similar durations, but with 1.25-fold increase in Ca 2+ concentrations at Shigella -invasion sites. Thus, the value of the diffusion coefficient in the actin focus controls both the amplitude of the Ca 2+ increase and the delay between invasion and RATP occurrence. These results, taking into account diffusion parameters falling in the range of what we experimentally determined for small molecules at invasion sites, are in line with the amplitude of RATPs experimentally observed during Shigella invasion. An interesting prediction of the computer simulations is that both inhomogeneities in InsP 3 and InsP 3 Rs levels in the actin foci need to be linked to get the localized sustained Ca 2+ responses. Indeed, if diffusion was not restricted ( Fig. 4f , inset), no significant local Ca 2+ increase was observed. INTs and diffusion in Shigella ipaA -mutant actin foci We then wanted to test the predicition of our model establishing a critical role of the actin meshwork-based diffusion restriction on the elicitation of RATPs at bacterial invasion sites. For this, cells were challenged with an ipaA mutant, which induces actin foci at the same frequency than wild-type Shigella , but fails to organize a dense actin meshwork in close apposition to bacteria and invades cell inefficiently [8] , [9] ( Fig. 3e ). Consistent with an absence of role of IpaA in the initial steps of invasion leading to bacterially induced actin polymerization, InsP 3 and InsP 3 Rs were osberved to accumulate at actin foci induced by an ipaA mutant to a similar extent than in foci induced by wild-type Shigella ( Fig. 4a and Supplementary Fig. S11 ). Remarkably, however, FRAP analysis indicated that foci induced by the ipaA mutant showed faster diffusion rates than those induced by wild-type Shigella , with an average t 1/2 =247±13 ms (61 foci, N =4). Because the effects of IpaA on actin reorganization at Shigella -invasion sites are mediated by its ability to bind to and to activate the focal adhesion protein vinculin, permitting the remodelling of actin filaments at bacterial invasion sites, these results further support the notion that actin filaments’ organization restricted diffusion at Shigella entry sites. Consistent with the notion that the restriction of diffusion at bacterial entry sites is critical for the duration of local Ca 2+ responses, the ipaA mutant induced less INTs than wild-type Shigella , and virtually no RATPs ( Fig. 1f ). The recruitment of InsP 3 R1 and GFP-PHPLC-δ1 in foci induced by the ipaA mutant at levels comparable to foci induced by wild-type Shigella suggested that the absence of RATPs in this mutant was linked to an altered actin meshwork and faster diffusion at the invasion sites ( Fig. 4a ), a situation that corresponds to the simulation shown in the inset of Fig. 4f . Mitochondrial activation at bacterial entry sites Because Ca 2+ is a key regulator of mitochondrial functions, we next wanted to test the consequences of RATPs on mitochondrial activation during Shigella invasion [34] , [35] . Although Ca 2+ transients activate mitochondrial ATP synthesis, sustained mitochondrial Ca 2+ increases lead to the loss of mitochondrial membranes integrity and the release of pro-apoptotic factors and cell death [35] . Interestingly, following prolonged incubation for several hours and intracellular multiplication, Shigella was shown to induce a necrotic-like cell death, linked to global Ca 2+ influx and mitochondrial damage [36] . As shown in Fig. 5 , mitochondria could be detected early during bacterial invasion, in Shigella -induced actin foci. Mitochondria were detected in all foci analysed, either at the close vicinity of invading bacteria or trapped in the actin meshwork induced by wild-type Shigella or the ipaA mutant ( Fig. 5a ). Confocal fluorescence microscopy analysis, however, indicated that InsP 3 R1 labelling in bacterially induced actin foci did not co-localize with mitochondria, suggesting that their presence implicated distinct processes ( Supplementary Fig. S14 ). An expected consequence of RATPs would be a sustained activation of mitochondria at invasion sites. Mitochondria were detected at bacterial invasion sites, entrapped in bacterially induced polymerized actin ( Fig. 5a ). To follow changes in mitochondrial Ca 2+ (Ca 2+ mito ), cells were transfected with the fluorescence resonance energy transfer (FRET)-based sensor 4mtD3cpV [37] . Upon challenge with Shigella , an increase in Ca 2+ mito was observed in 94±9% of the foci analysed (35 foci, N =7). Moreover, as illustrated in Fig. 5 , Ca 2+ mito increases at entry sites could occur independent of variations of Ca 2+ mito in the rest of the cell, and like RATPs, could last several tens of seconds ( Fig. 5c ). When cells were challenged with the ipaA mutant, however, only 42±11% of bacterially induced foci were associated with an increase in Ca 2+ mito (31 foci, N =5). Furthermore, foci induced by the ipaA strain were seldom associated with long-lasting Ca 2+ mito increases, consistent with the low frequency of RATPs induced by this mutant ( Fig. 5d ). 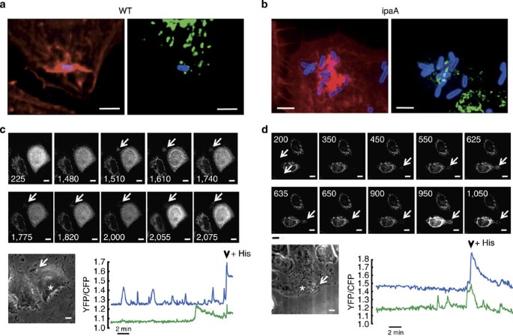Figure 5: Mitochondrial activation duringShigellainvasion. Staining of F-actin (red) and bacterial lipopolysaccharide (blue) of cells transfected with 4mitD3cpv (green) challenged with wild-type (WT) (a) oripaA-mutantShigella(b). (c,d) Ratio images of citrine (YFP)/Cyan Fluorescent protein (CFP) emissions in time-lapse analysis of 4mitD3cpv-transfected cells challenged with WTShigella(c) or theipaAmutant (d). Time after challenge in ms. Arrows: invasion foci. Scale bar, 5 μm. Traces: average intensity in invasion foci (green) or control area (blue). Arrowheads: addition of 20 μM histamine (His). Figure 5: Mitochondrial activation during Shigella invasion. Staining of F-actin (red) and bacterial lipopolysaccharide (blue) of cells transfected with 4mitD3cpv (green) challenged with wild-type (WT) ( a ) or ipaA -mutant Shigella ( b ). ( c , d ) Ratio images of citrine (YFP)/Cyan Fluorescent protein (CFP) emissions in time-lapse analysis of 4mitD3cpv-transfected cells challenged with WT Shigella ( c ) or the ipaA mutant ( d ). Time after challenge in ms. Arrows: invasion foci. Scale bar, 5 μm. Traces: average intensity in invasion foci (green) or control area (blue). Arrowheads: addition of 20 μM histamine (His). Full size image As opposed to long-term bacterial infection, however, mitochondrial swelling could be not detected at early time points of infection [36] , suggesting that local and prolonged increases in mitochondrial Ca 2+ did not induce mitochondrial dysfunction. To confirm this, we used the F 1 /F 0 ATP synthase inhibitor oligomycin A [38] to determine the contribution of mitochondrial ATP in our experimental conditions. Dosage of cytosolic ATP levels indicated that mitochondrial ATP synthase activity accounted for 85% of the total ATP levels ( Supplementary Fig. S15 ). Furthermore, Shigella invasion resulted in a 10–20% depletion of global ATP pools, indicating that bacterial invasion did not result in a general mitochondrial dysfunction ( Supplementary Fig. S15 ). These results are in line with the notion that the confinement of sustained local Ca 2+ responses allow the prolonged activation of mitochondria at invasion sites. To enter efficiently into cells, Shigella needs to establish a dense meshwork of actin filaments at the plasma membrane–bacterial contact site, which is allowed by the vinculin-binding type III effector IpaA. Here we bring evidence that this actin meshwork limits diffusion of free solutes, probably by creating mechanical obstructions as reported in other systems [29] , [30] . We propose that during Shigella invasion, the local activation of PLC-β1 and -δ1 leads to accumulation of InsP 3 at invasion sites ( Supplementary Fig. S16 ). InsP 3 Rs enriched at bacterially induced actin foci, possibly through a diffusion-capture process involving InsP 3 binding or through interaction with a cytoskeletal protein such as band 4.1 (ref. 39 ), shown critical for bacterial invasion. Previous studies have reported that Puffs elicited by InsP 3 (ref. 40 ) stimulation could originate from pre-clustered InsP3Rs, or alternatively, implicated the de novo clustering of InsP 3 Rs [41] . Although we observed Puff-like responses elicited early upon bacterial challenge, these did not appear specific for bacterial invasion. In contrast, RATPs at bacterially induced foci were associated with a massive recruitment of InsP 3 Rs, which could either result from InsP 3 -mediated clustering of InsP 3 Rs or, given the extended kinetics of the invasion process, possibly through the recruitment of pre-clustered InsP 3 Rs at Shigella -invasion sites. As modelled in this study, restricted diffusion is critical for the elicitation of sustained local Ca 2+ increases at entry sites ( Supplementary Fig. S16 ). There are multiple implications of long-lasting local Ca 2+ responses during Shigella invasion. RATPs will regulate the function of Ca 2+ -dependent enzymes, which may have an impact on cytoskeletal reorganization at the site of bacterial invasion. For example, calpains, whose proteolytic activity is Ca 2+ dependent, have been implicated in Shigella invasion [42] . Also, myosin II, whose activity is regulated by Ca 2+ , has been implicated in Salmonella invasion, a process sharing similarities with Shigella invasion [43] . The confinement of RATPs at invasion sites may also allow to limit the spreading of apoptotic signals linked to prolonged elevated mitochondrial Ca 2+ during the early stages of infection. Mitochondrial activation through InsP 3 -mediated Ca 2+ increase allows ATP production through oxidative phosphorylation [34] . Interestingly, local ATP supply was shown critical for cytoskeletal remodelling processes requiring high energy during phagocytosis, a process sharing similarities with Shigella invasion [44] . In future work, it will be interesting to determine if mitochondria favour bacterial invasion, by allowing the local production of ATP required for elongation of actin filaments. Antibodies and reagents The rabbit polyclonal antibody against the type 1 InsP3 receptor (ABR Affinity Bioreagents) and the mouse monoclonal antibody against type 3 InsP 3 receptor (Transduction laboratories) were both used at a dilution of 1:1,000 and 1:100 for western blot and immunofluorescence analysis, respectively. The sarco/endoplasmic reticulum Ca 2+ -ATPase (SERCA) inhibitor tBuBHQ, the F-actin inibitors cytochalasin D and latrunculin B were from Sigma-Aldrich. The anti-lipopolysaccharide polyclonal Ab was described previously and was used at a 1:1000 dilution [28] . γ-(6-Aminohexyl)-ATP-Atto488 (fATP) was from Jena Biosciences. Calcein-AM, FITC-dextrans (3 and 10 kDa), Phallicidin-A488, anti-rabbit IgG-A547 and the fluorescent Ca 2+ probes, Fluo-4-AM, Fura-Red-AM and Fura-2-AM, were from Invitrogen Corp. siRNAs against the type 1 and type 3 InsP 3 receptors were from Qiagen. Cell lines, bacterial strains and plasmids The wild type Shigella serotype V M90T and its isogenic derivatives mxiD and ipaA were described previously [45] . Bacteria were grown in trypticase Soy broth at 37 °C in a shaking incubator. HeLa cells were from ATCC. HCx26 cells were described previously [3] . All cells were grown in RPMI medium containing 5% fetal calf serum in a 5% CO 2 incubator. The plasmid encoding the genetically encoded mitochondrial Ca 2+ FRET sensor 4mitD3cpv was described previously [46] . The gene encoding the type I InsP 3 -5′ phosphatase was retrieved by Kpn I and Eco RV digestion from the previously described clone D1 [25] and subcloned, after a T4 DNA polymerase treatment into the pIRES-GFP vector (Clontech) using the Eco 47III restriction enzymes to generate pIRES-InsP 3 -5P-GFP. Constructs were checked by DNA sequencing. Cells were transfected with plasmid constructs using JetPei (Polyplus) or with anti-InsP 3 R siRNA using the HiPerfect transfection reagents (Invitrogen) following the manufacturer’s instructions. Immmunofluorescence analysis of Shigella -induced actin foci Shigella -induced actin foci of invasion were scored as described previously [6] . When mentionned oligomycin A was added at a final concentration of 5 or 10 μg ml −1 for 16 h at 37 °C before bacterial challenge. Statistical analysis For all samples, significance relative to control samples was tested using an unpaired Student’s t- test with unequal variance unless otherwise stated. Calcium fluorescence microscopy imaging Analysis of global Ca 2+ variations was performed by loading cells with 3 μM Fura-2-AM in EM buffer containing 120 mM NaCl, 7 mM KCl, 1.8 mM CaCl2, 0.8 mM MgCl2, 5 mM glucose and 25 mM HEPES pH 7.3, as described previously [3] . For high-speed analysis of local Ca 2+ variations, cells were loaded with 3 μM Fluo-4-AM. Samples were analysed at 33 °C on an inverted Leica DMRIBe fluorescence microscope, equiped with light-emitting diode 470 nm illuminating sources and a 480 nm band pass excitation filter, a 505 nm dichroic filter and a 527-band pass emission filter driven by the Metamorph software from Roper Scientific Instruments. Images were captured using a Cascade 512B EM-CCD back-illuminated camera in a stream mode, with an acquisition every 30 ms. Changes in the ratio of Fura-2 (Δ R ) or Fluo-4 fluorescence intensity (ΔF) were calculated relative to the resting ratio or fluorescence value ( R 0 or F 0 ) as Δ R / R 0 or ΔF/F 0 , respectively. Cells showing local Ca 2+ responses were scored by High Speed Fluorescence Microscopy (HSFM). The average percentage of responsive cells showing at least a detectable Ca 2+ response during the length of the analysis was determined. The amplitude of local responses corresponded on average to 6.9±0.6 ( N =16) and 55±6% ( N =12) of the maximal response obtained using histamine as an agonist at the maximal concentration of 30 μM, for puff-like and RATP responses, respectively. To monitor variations in mitochondrial Ca 2+ , cells transfected with the 4mitD3cpv construct were analysed using a dichroic 455DRLP, and the following filters: 450 nm excitation and 490 nm emission filters for cyan fluorescent protein (CFP), 490/40 nm excitation and 535/40 nm emission filters for citrine, and 450 nm excitation and 535/40 nm emission filters for the FRET image. All images were corrected for background fluorescence. Calcein loading and FRAP analysis Cells grown on cover slips were loaded with 3 μM calcein-AM by incubation in EM buffer or, alternatively, by microelectroporation for fATP, 3 kDa- and 10 kDa dextran-FITC ( Supplementary Information ). Samples were mounted in an observation chamber on a plate heated at 37 °C on an inverted spinning disk confocal microscope (Nikon Eclipse Ti) analysed with a × 60 objective lens, using an EM-CCD camera Evolve equipped with a FRAP module and driven by the Metamorph software (Roper Scientific Instruments), allowing the acquisition of images during the bleaching phase. Samples were challenged with Shigella strains at a multiplicity of infection of 5–10 (final OD 600nm =0.1) for 15 min. For each samples, bleaching and image acquisition were performed using identical conditions, with the exception of the bleach area defined to encompass bacterial invasion foci. Variations in the bleach area size, however, did not exceed 10% between all samples. An area of an average size±s.e.m. of 24.2±0.7 μm 2 , corresponding to the bacterial invasion foci, was bleached using a 470 nm excitation laser for 80 ms until fluorescence was reduced to background levels. For each experiment, an area identical to the bacterial foci area was bleached in another cell in the same field. Image acquisition was performed under the stream mode every 30 ms, with 200 frames during pre-bleach and 2,000 frames to monitor fluorescence recovery. Relative fluorescence intensity was determined as FRAP%=(F t /C t )/ (F 0 / C 0 ) × 100, where F 0 and C 0 represent the intensity of the bleached and control unbleached regions, respectively, before bleaching, and F t and C t represent the intensity at time t after bleaching for the same corresponding regions. Fluorescence recovery curves corresponding to the normalized intensity in the bleached area averaged from several measurements showed good quality fit with a single-component diffusion (>32 foci, N =6). Immunofluorescence staining Immunofluorescence analysis was performed as described previously [7] . Stacks of focal planes spaced by 0.2 μm were processed for point spread function (PSF)-based three-dimensional deconvolution in the Metamorph software 7 or 4 (Universal Imaging) using a fast algorithm. Reconstructions were obtained by applying the average function on the stacks of deconvolved images. Modelling The site of bacterial invasion, modelled as a 5 × 5 μm 2 region located at the upper, central part or the cell, shows reduced diffusibility, with InsP 3 and Ca 2+ diffusion coefficients 1.6 times smaller than that in the rest of the cytoplasm, and increased density of InsP 3 Rs (three times higher than in the rest of the cytoplasm). If diffusion is restricted, but without increased density of InsP 3 Rs, no increase in Ca 2+ is observed (not shown). Figure 4e has been obtained by numerical integration of three differential equations, simulating the evolution of the fraction of inhibited InsP 3 receptors ( R i ), the concentration of cytosolic Ca 2+ ( C ) and the concentration of InsP 3 ( I ): where represents the fraction of open receptors. Equation (1) reflects the activation/inhibition of the InsP 3 R by cytosolic Ca 2+ . Equation (2) describes changes in cytosolic Ca 2+ concentration due to Ca 2+ release from the endoplasmic reticulum assumed to remain constant, uptake through the SERCA pumps and diffusion. Equations (1) and (2) are based on Dupont and Swillens [32] and represent a classical description of Ca 2+ dynamics [47] . Equation (3) is a simplified description of intracellular InsP 3 dynamics, taking into account synthesis through PLC at a basal rate ( V b ), localized stimulated synthesis due to bacterial invasion ( J IP ), linear degradation ( k d I ) and diffusion. These equations have been integrated with MatLab (ode23) in two dimensions, using a 60 × 24 mesh to simulate the dynamics occurring in a 25 × 10-μm cell. The geometry of the system is schematized in Supplementary Fig. S12 . The parameters are defined in Supplementary Table S1 . Initial conditions correspond to the steady-state situation in the absence of bacterial invasion (see Supplementary Methods for more detailed information). How to cite this article: Tran Van Nhieu, G. et al. Actin-based confinement of calcium responses during Shigella invasion. Nat. Commun. 4:1567 doi: 10.1038/ncomms2561 (2013).